Universal composition–structure–property maps for natural and biomimetic platelet–matrix composites and stacked heterostructures Many natural and biomimetic platelet–matrix composites—such as nacre, silk, and clay-polymer—exhibit a remarkable balance of strength, toughness and/or stiffness, which call for a universal measure to quantify this outstanding feature given the structure and material characteristics of the constituents. Analogously, there is an urgent need to quantify the mechanics of emerging electronic and photonic systems such as stacked heterostructures. Here we report the development of a unified framework to construct universal composition–structure–property diagrams that decode the interplay between various geometries and inherent material features in both platelet–matrix composites and stacked heterostructures. We study the effects of elastic and elastic-perfectly plastic matrices, overlap offset ratio and the competing mechanisms of platelet versus matrix failures. Validated by several 3D-printed specimens and a wide range of natural and synthetic materials across scales, the proposed universally valid diagrams have important implications for science-based engineering of numerous platelet–matrix composites and stacked heterostructures. Natural materials such as nacre, spider silk, tendon and so on are primarily biocomposites that exhibit an excellent balance of mechanical properties and multi-functionality far beyond their constituents [1] , [2] . For instance, nacre is made of 95% aragonite, a brittle mineral, but demonstrates a toughness that is ~3,000 times larger than aragonite with the expense of minor reduction in stiffness [3] . The key to success of these biocomposites is their nano/micrometre-size building blocks, which consist of hard inorganic platelets connected by a soft organic matrix in a brick-and-mortar pattern, known as platelet–matrix composites [4] , [5] . Numerous efforts are reported to decode the complexities and synergies behind the interacting constituents of natural and biological platelet–matrix composites with the goal of fabricating similar synthetic composites [6] , [7] , [8] , [9] , [10] , [11] , [12] . In this context, application of the well-known ‘shear-lag’ model [13] , [14] has proven to be essential in theoretically advancing the knowledge of load transfer in collagen fibrils [15] , nacre [16] and nanotube-reinforced polymer composites [17] to name a few. For instance, Zhang et al . [18] studied mechanical properties of elastic platelet–matrix composites with different platelet distributions. With the assumption of uniform shear stress distribution, a critical platelet aspect ratio was reported that distinguishes the platelet versus matrix failures. Begley et al . [19] lifted the assumption of uniform shear stress and introduced different failure mechanisms for composites with a plastic matrix and uniform distribution of identical platelets. More recent studies proposed characteristic overlap lengths for elastic and plastic composites with uniform distribution of identical platelets [20] . Overall, given the material heterogeneity and structural variety of numerous natural and biomimetic platelet–matrix composites, there is currently no unified understanding of the interplay between various geometers and inherent material characteristics in controlling the balance of mechanical properties. The latter is essentially unexplored for composites made of dissimilar platelets. A prime example of such composites are stacked heterostructures in emerging electronic and photonic devices that are made of alternating two-dimensional (2D) sheets of nanometre size connected by a network of weak van der Waals [21] , [22] , [23] , [24] or covalent bonds [25] representing the soft matrix [22] ( Fig. 1b ). For example, field-effect tunnelling transistors with high On/Off ratios were recently fabricated by graphene (G) heterostructures sandwiching atomically thin hexagonal boron nitride (h-BN) or molybdenum disulfide (MoS 2 ) sheets acting as a vertical transport barrier [21] . Similarly, h-BN/G/h-BN layers were fabricated as electronic devices with high cutoff frequency [24] and potentially tunable and sizable bandgap via aligning G and h-BN in various ways [26] . Controlling the nanoscale mechanical properties of stacked heterostructures is a fundamentally significant and challenging topic, which remains largely unexplored [27] . 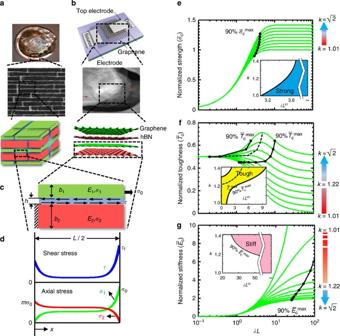Figure 1: Mechanical properties in elastic platelet–matrix composites. (a) Structure of nacre along with a schematic model (adapted with permission from20. Copyright 2012 American Chemical Society). (b) A cartoon of a 2D-stacked heterostructures along (adapted with permission from ref.22) with a transmission electron microscope image of 2D alternating h-BN and graphene sheets (adapted with permission from ref.23Copyright 2012 American Chemical Society). (c) A 2D unit cell of the composites ina,bmade of two platelets connected by a matrix (blue). (d) typical asymmetrical and non-uniform shear and axial stress distributions along the overlap length of the unit cell in (c). The top platelet is assumed to be softer than the bottom one. (e–g), Normalized strength,, toughness,, and stiffness,, of the unit cell incas a function ofλLandk. To avoid singularity,kstarts from 1.01 (e) the solid black circles denotes the points wherebecomes 90%for eachk. The inset represents the ‘strong’ region in the space of (λL,k). Owing to strength normalization toλ, this parameter (λ) is constant in the horizontal axis and only the overlap length,L, is the varying parameter. (f) The dashed and solid lines show the points ofand 90%, respectively. The inset represents the ‘tough’ region in the space of (λL,k). (g) The black line denotes the points wherebecomes 90%. The inset represents ‘stiff’ region based on. Figure 1: Mechanical properties in elastic platelet–matrix composites. ( a ) Structure of nacre along with a schematic model (adapted with permission from [20] . Copyright 2012 American Chemical Society). ( b ) A cartoon of a 2D-stacked heterostructures along (adapted with permission from ref. 22 ) with a transmission electron microscope image of 2D alternating h-BN and graphene sheets (adapted with permission from ref. 23 Copyright 2012 American Chemical Society). ( c ) A 2D unit cell of the composites in a , b made of two platelets connected by a matrix (blue). ( d ) typical asymmetrical and non-uniform shear and axial stress distributions along the overlap length of the unit cell in ( c ). The top platelet is assumed to be softer than the bottom one. ( e – g ), Normalized strength, , toughness, , and stiffness, , of the unit cell in c as a function of λL and k . To avoid singularity, k starts from 1.01 ( e ) the solid black circles denotes the points where becomes 90% for each k . The inset represents the ‘strong’ region in the space of ( λL , k ). Owing to strength normalization to λ , this parameter ( λ ) is constant in the horizontal axis and only the overlap length, L , is the varying parameter. ( f ) The dashed and solid lines show the points of and 90% , respectively. The inset represents the ‘tough’ region in the space of ( λL , k ). ( g ) The black line denotes the points where becomes 90% . The inset represents ‘stiff’ region based on . Full size image Here we facilitate a comprehensive understanding of the mechanics of platelet–matrix composites and stacked heterostructures in the shear mode via universal composition–structure–property maps. By considering both elastic and elastic-perfectly plastic matrices as well as platelets with offset overlap ratios, we identify a universal dimensionless characteristic quadruple, ( λL , k , C , ξ ), which governs the mechanical properties (stiffness, strength and toughness) of the platelet–matrix composites and stacked heterostructures consisting of both similar and dissimilar platelets. Next, via mapping an extensive spectra of ( λL , k , C , ξ ) parameters into a set of 2D diagrams, we unify and infer important composition–structure–property relationships in platelet–matrix composites. The universality of the these diagrams will be compared with a series of three-dimensional (3D)-printed specimens, and a wide range of existing natural and biomimetic platelet–matrix composites as well as stacked heterostructures across several length scales and material classes. Finally, we will study and compare the competing mechanisms between platelet and matrix failures as well as the failure of platelet–matrix composites with stairwise and random staggering architectures. Elastic matrix with no overlap offset The dominant deformation mechanism of both platelet–matrix composite such as nacre ( Fig. 1a ) or a stacked heterostructure such as h-BN-graphene ( Fig. 1b ) [23] can be represented by a 2D unit cell under shear loading as shown in Fig. 1c . In view of this common building block, hereto we refer to ‘generalized platelet–matrix composite’ as an archetype composite consisting of both conventional platelet–matrix composites and stacked heterostructures. First, we focus on elastic composites ( C =0) with varying platelet dissimilarity ( k ) and no overlap offset ( ξ =0.5). Then, the results will be extended to composites with elastic-perfectly plastic matrices and platelets with varying overlap offset ratios (varying C and ξ). The 2D model of the generalized platelet–matrix composite is made of two platelets with Young’s moduli, E 1 and E 2 and widths of b 1 and b 2 , and is subjected to stress σ 0 on the right end of the top platelet. In addition, the system is clamped at the left end of the bottom platelet and traction free on all other dimensions except the overlap length, L /2. The two platelets are connected by a thin film (matrix) with shear modulus G and thickness h . For a unit lateral dimension, the elastic stress distributions to this system are [28] In equation (1), σ 1 and σ 2 are the axial stresses on the top and bottom platelets, respectively, τ is the shear stress between the two platelets, m = b 1 / b 2 and n = E 1 / E 2 are the ratios of the widths and Young’s moduli of the two platelets, is a unified parameter representing both the geometrical and elastic contrast of the two platelets and is a normalized parameter denoting the interface properties (shear modulus and thickness). The above elastic solutions generalizes the common shear-lag problem [14] , [20] , [29] to non-identical platelets and dimensions. In equation (1), λkL is a key dimensionless parameter encompassing all the structural and elastic material information of the generalized platelet–matrix composites with similar or dissimilar platelets. This parameter can be deconvoluted into two dimensionless parameters, λL and k , which control, respectively, the (non)uniformity and (a)symmetry of the elastic stress distributions ( Fig. 1d ). A small (large) λL corresponds to more uniform (non-uniform) shear stress distribution in the matrix and linear (non-linear) axial stresses in the platelets ( Fig. 2 ). For identical platelets (that is, mn =1 and thus ), equation (1) represent symmetric stress distributions with respect to L /4. For dissimilar platelets, that is, , equation (1) demonstrate asymmetrical stress distributions ( Fig. 1d and Fig. 2 ). However, for varying m and n ratios, as long as the product of mn (or k ) is constant, all the shear and axial stress distributions (equation (1)) remain unchanged. This concept is similar to the notion of ‘transformed area’ in homogenizing the composite behaviour of materials where both width and Young’s modulus can be used interchangeably (with proper factors) [30] . Together the extent of the aforementioned asymmetry and non-uniformity in stress distributions govern key mechanical properties, such as strength, toughness and stiffness, of the platelet–matrix composite. This will be discussed in the next section. 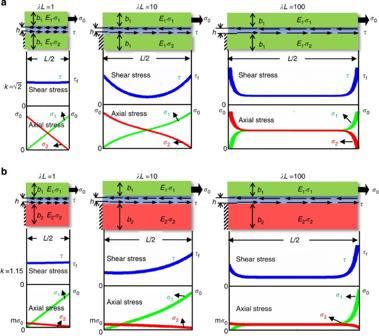Figure 2: Influence ofλLandkon uniformity and symmetry of stress distributions. (a)λLincreases from left to right in platelet–matrix composites made of similar and (b) dissimilar platelets. From left to right, uniform shear stress changes to non-uniform stresses along the overlap length, and the linear axial stresses to non-linear stresses. This observation is valid for both (a,b) cases, corresponding to composites ofand dissimilar platelets (k=1.15). Analogously, by changing the dimensionless parameterk, fromto 1.15, we notice how stresses change from symmetric to asymmetric distributions along the overlap length. This observation is valid for all ranges ofλL. Figure 2: Influence of λL and k on uniformity and symmetry of stress distributions. ( a ) λL increases from left to right in platelet–matrix composites made of similar and ( b ) dissimilar platelets. From left to right, uniform shear stress changes to non-uniform stresses along the overlap length, and the linear axial stresses to non-linear stresses. This observation is valid for both ( a , b ) cases, corresponding to composites of and dissimilar platelets ( k =1.15). Analogously, by changing the dimensionless parameter k , from to 1.15, we notice how stresses change from symmetric to asymmetric distributions along the overlap length. This observation is valid for all ranges of λL . Full size image Strength To understand the strength behaviour of the unit cell in Fig. 1c , we note that by increasing the applied stress, σ 0 , the average shear stress, , increases to satisfy the force equilibrium, σ 0 b 1 =0.5 τ ave L , until the shear stress reaches the maximum shear strength, τ f , assuming the platelets are strong enough such that the composite fails in the shear mode (the case of platelet failures will be discussed later). When mn <1 (for example, top platelet is softer than the bottom one), the maximum shear stress occurs at x = L /2 ( Fig. 1d ), and when mn >1, the maximum shear stress occurs at x =0. Without loss of generality, we consider mn <1, and thus throughout this work. In this case, τ f reads where is the ultimate axial stress that can be applied to the top platelet preceding interface failure at τ f . By rearranging equation (2) and use of the relation, , the effective strength of the unit cell on interface failure becomes where A ( L )=coth ( λkL /2)+( k 2 −1)csch( λkL /2) and B = b 1 + b 2 + h . Figure 1e shows the normalized dimensionless strength, , of the unit cell for varying characteristic overlap lengths, λL , and a range of platelet contrasts between two extremes, that is, k =1 (dissimilar platelets) and (identical platelets). By increasing k from 1 to (reducing platelet dissimilarity), normalized strength increases for large λL . This pattern indicates that the use of identical platelets maximizes the strength capacity. Furthermore, for all values of k , the normalized strength asymptotically saturates with λL to the upper limit of strength for elastic composites under matrix failure, that is, . Toughness Toughness is a crucial property for functionality of several natural and synthetic platelet–matrix composites [7] , [11] . It is defined as the amount of energy per volume a material absorbs before it fails [2] . Although related, this definition is different than the classical definition of ‘fracture toughness’ with the unit of . While many toughening mechanisms in natural materials take place during crack propagations and/or interlocking mechanisms (so-called extrinsic mechanisms [31] ), here we focus on toughening mechanisms associated with the strain energy density of the system, that is, intrinsic mechanisms. For a linear generalized platelet–matrix composite in Fig. 1c (linear elastic platelets and elastic matrix) toughness reads By substituting equation (1) into equation (4), taking the integrals and using of equation (2) for , we obtain where D ( L )=[ k 4 coth ( λkL /2)+( k 2 −1)( λkL /2−2 tan h ( λkL /4))]/( λkL ). For any given , Fig. 1f demonstrates the variation of normalized toughness, , as a function of λL . As illustrated in this figure, for a limited range of k , , has optimum values at certain λL , with (identical platelets) having the maximum (see dashed lines). For other values (1< k <1.2247), the maximum occurs at the limit of λL →0, which is not practical; hence for any finite λL the actual toughness is smaller than the maximum capacity. Interestingly, k =1.2247 exactly corresponds to mn =0.5. Therefore, the generalized platelet–matrix composites whose platelets have a stiffness ratio or a width ratio of more than 2, or the combination thereof such that mn <0.5, do not have an optimum toughness. Thus, such composites cannot exhibit a high toughness when compared with those with . Furthermore, when λL →∞, all values reduce to an asymptotic level of ( k 2 −1)/2, indicating that toughness becomes vanishingly small for composites made of completely dissimilar platelets, that is, k →1. Stiffness An effective Young’s modulus, E c , representing the stiffness of the generalized platelet–matrix composite, can be calculated from . Thus, in view of equations (3) and (5), E c becomes Figure 1g shows the normalized stiffness, , versus λL , which eventually saturates to . For composites with continuous platelets, is equal to the average stiffness of the platelets. Note that this figure may imply that identical platelets result in lower stiffness. However, this is due to normalization to E 1 , which is considered to be the softer platelet in this study. Indeed, for a unit cell to offer its maximum stiffness capacity, both platelets must be as stiff as possible. Experimental validations To validate the above theoretical elastic derivations, we performed tensile tests on a series of 3D-printed though-model specimens made of distinct platelets and matrices. We fabricated twelve prototypes with a wide range of overlap lengths, width ratios and three distinct materials, that is, A, B and C. (see Fig. 3 , Supplementary Figs 1–3 , Supplementary Table 1 , and Supplementary Methods ). To have a comparative advantage, all the specimens are grouped as ( a,a′ ), ( b,b′ ), ( c,c′ ), ( d,d′ ), ( e,e′ ), ( f,f′ ) where within each group λL is identical, but k takes the value of either for specimens with identical platelets, or 1.155 for specimens with dissimilar platelets symbolized by the prime notations. 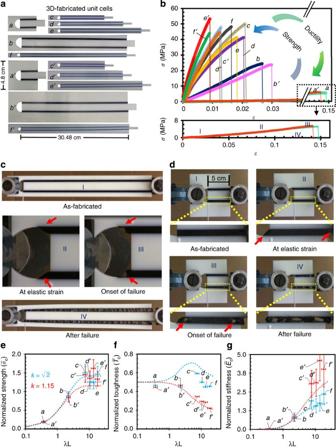Figure 3: Tensile experiments on 3D-fabricated specimens made of similar and dissimilar platelets. (a) Planar representation of 12 3D-printed specimens. Specimensa–fare made of similar plateletswhile specimensa′–f′are made of dissimilar platelets (k=1.15). In each group, the platelet–matrix materials are distinct. (b) The measured effective stress–strain plots of the specimens ina. The inset shows the zoom-in plots of the specimensaanda′, which exhibit significant ductility. (c,d) Typical snapshots of the pre-and post-failure during tensile experiments. The arrows indicate the locations of maximum shear stresses. (c) Refers to the specimenbrepresenting a unit cell with similar platelets and (d) refers to the specimena′ representing a unit cell with dissimilar platelets. (e–g) normalized strength, toughness and stiffness of the specimens inaversus characteristic overlap lengthλL. For comparison, theoretical predictions (dashed lines) are also given. The error bars are due to uncertainty in the Young modulus of the base material (E1), which corresponding changeλ(horizontal error bars) and normalization factors (vertical error bars). The normalization factor ofdoes not depend onE1. Figure 3b shows the measured stress–strain plots of all specimens. Details of pre-failure and post failure of two representative specimens made of similar and dissimilar platelets are depicted in Fig. 3c,d . On straining, the as-fabricated unit cells (snapshot I), the platelets undergo elastic deformations, while the interface undergoes large shear deformation (snapshot II), owing to the soft material phase of the matrix ( Supplementary Movie 1 ). Snapshot III demonstrates the onset of failure, which starts form the two extreme ends due to the larger shear stresses at these points (see, for example, Fig. 1d ). Finally, the large shear stresses rapidly cover the entire overlap length and the unit cell fails (snapshot IV). Figure 3: Tensile experiments on 3D-fabricated specimens made of similar and dissimilar platelets. ( a ) Planar representation of 12 3D-printed specimens. Specimens a – f are made of similar platelets while specimens a′ – f′ are made of dissimilar platelets ( k =1.15). In each group, the platelet–matrix materials are distinct. ( b ) The measured effective stress–strain plots of the specimens in a . The inset shows the zoom-in plots of the specimens a and a ′, which exhibit significant ductility. ( c , d ) Typical snapshots of the pre-and post-failure during tensile experiments. The arrows indicate the locations of maximum shear stresses. ( c ) Refers to the specimen b representing a unit cell with similar platelets and ( d ) refers to the specimen a ′ representing a unit cell with dissimilar platelets. ( e – g ) normalized strength, toughness and stiffness of the specimens in a versus characteristic overlap length λL . For comparison, theoretical predictions (dashed lines) are also given. The error bars are due to uncertainty in the Young modulus of the base material ( E 1 ), which corresponding change λ (horizontal error bars) and normalization factors (vertical error bars). The normalization factor of does not depend on E 1 . Full size image Figure 3e–g shows the measured strength, toughness and stiffness, which are extracted from Fig. 3b , and are normalized using factors identical to those detailed above ( Supplementary Tables 2 and 3 ). The general trends and magnitude of these normalized experimental values match very well with those of theoretical predictions (dashed lines). Elastic-perfectly plastic matrix with no overlap offset In many natural and synthetic platelet–matrix composites, the matrix is highly ductile and can undergo large plastic deformation. Here plasticity is introduced by considering an elastic-perfectly plastic matrix with a dimensionless parameter , representing the degree of matrix plasticity where γ y denotes the yielding strain and γ f represents the final strain of the matrix preceding the failure. While the detailed calculations for the modified strength and toughness are provided in the Supplementary Note 4 (stiffness is identical to that of elastic solution), in essence, the matrix plasticity and dissimilarity of the platelets results in three distinct failure mechanisms depending on geometry and material properties: case 1) failure occurs at the right side, that is, γ ( x = L /2)= γ f , before the left side reaches the yielding shear strain, γ ( x =0)< γ y ; therefore, there exists one plastic zone at the right side and one elastic zone (the rest) at the left side, case 2) failure occurs at γ ( x = L /2)= γ f and the left side enters the plastic regime but never fails before the right side, that is, γ y < γ ( x =0)< γ f , while an elastic zone is present at the middle. Therefore, there are two plastic zones at the two ends and one elastic zone in the middle and case 3) failure occurs at γ ( x = L /2)= γ f when the whole overlap length enters the plastic regime, that is, γ y < γ ( x < L /2)< γ f . Note that in the latter case, although the shear stress in the full overlap length is constant and equal to τ f , the shear strain γ has a non-linear distribution across the overlap length ( Fig. 4 ). 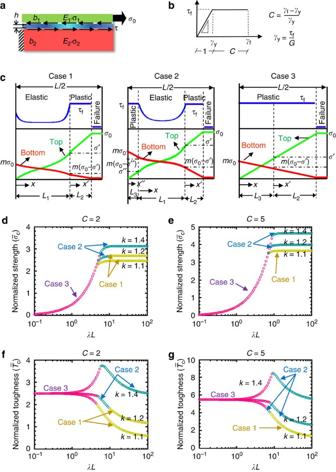Figure 4: Failure mechanisms and mechanical properties for composites with plastic matrix. (a) Schematic view of a unit cell exhibiting tensile stress on the platelets and shear stress in the matrix. (b) Plasticity in the matrix is considered using an elastic-perfectly plastic shear deformation model. The parameterCrepresents the degree of plasticity, which is the ratio of the extra allowable strain of the matrix to the yielding strain. (c) Three different shear failure mechanisms are possible: case 1 with one elastic and one plastic region, case 2 with two plastic regions and one elastic region in the middle and case 3 where the full overall overlap length is in the plastic region. In all three cases, failure starts from the right end (free end of the stiffer platelet). (d,e) Normalized strength,, and (f,g) normalized toughness,, for two degrees of matrix plasticity,C=2 andC=5. Three values of dissimilarity ratios (k) are shown for eachC. The colour of the plots in denote different failure mechanisms occur at different overlap lengths,λL. Figure 4: Failure mechanisms and mechanical properties for composites with plastic matrix. ( a ) Schematic view of a unit cell exhibiting tensile stress on the platelets and shear stress in the matrix. ( b ) Plasticity in the matrix is considered using an elastic-perfectly plastic shear deformation model. The parameter C represents the degree of plasticity, which is the ratio of the extra allowable strain of the matrix to the yielding strain. ( c ) Three different shear failure mechanisms are possible: case 1 with one elastic and one plastic region, case 2 with two plastic regions and one elastic region in the middle and case 3 where the full overall overlap length is in the plastic region. In all three cases, failure starts from the right end (free end of the stiffer platelet). ( d , e ) Normalized strength, , and ( f , g ) normalized toughness, , for two degrees of matrix plasticity, C =2 and C =5. Three values of dissimilarity ratios ( k ) are shown for each C . The colour of the plots in denote different failure mechanisms occur at different overlap lengths, λL . Full size image Each case requires a distinct set of equations to calculate the lengths of the elastic and plastic regions to obtain the values of strength and toughness. However, regardless of the failure mechanism, it turns out that the behaviours of toughness and strength versus λL are similar to the fully elastic case, except that the ultimate values are increased by introduction of plasticity ( Supplementary Fig 4 and Fig. 5c–f ). 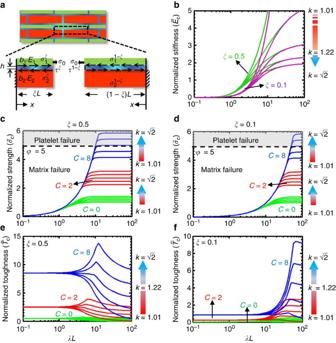Figure 5: Mechanical properties for composites with plastic matrix and overlap offset. (a) Schematic view of representative unit cell with non-uniform overlap (offset ratioξ). (b) Normalized stiffness,, is not a function ofCand is plotted for two values ofξ=0.5 andξ=0.1. (c,d), Normalized strength,, The dash lines correspond toϕ=5 as an example defining the boundary of platelet and matrix failures. (e,f), Normalized toughness,, are shown for varyingλL,kandC. Each colour represents a specificCandξbut varyingkfrom 1 to. Figure 5: Mechanical properties for composites with plastic matrix and overlap offset. ( a ) Schematic view of representative unit cell with non-uniform overlap (offset ratio ξ ). ( b ) Normalized stiffness, , is not a function of C and is plotted for two values of ξ =0.5 and ξ =0.1. ( c , d ), Normalized strength, , The dash lines correspond to ϕ =5 as an example defining the boundary of platelet and matrix failures. ( e , f ), Normalized toughness, , are shown for varying λL , k and C . Each colour represents a specific C and ξ but varying k from 1 to . Full size image Elastic-perfectly plastic matrix with overlap offset So far, all our results were based on platelets of length. L with an equal overlap length of L /2 on both sides, a so-called uniformly staggered distribution. Other staggering patterns are also observed in nature [15] . As a first step towards non-uniform platelet distributions, here we introduce a dimensionless parameter 0< ξ ≤0.5, denoting the overlap offset ratio between the platelets. In this case, the platelet length of L is divided into two parts of length ξL and (1– ξ ) L as shown in Fig. 5a . Equation (7) shows the derived strength, toughness and stiffness for any given quadruple of λL , k , C and ξ (see Supplementary Notes 5 and 6 for details): Here f σ , f T and f E are the dimensionless functions representing normalized strength, toughness and stiffness. Using ξ =0.5, equation (7) degenerates to a system with uniformly staggered distribution, and as ξ approaches zero the offset increases. Our analysis shows that for any triple of ( λL , k , C ), strength, toughness and stiffness are higher or equal (depending on λL ) in systems with ξ =0.5 than those with ξ <0.5, and they get lower as ξ →0 ( Fig. 5b–f ). Our results corroborate on the findings of Zhang et al . [18] (but further extend them to plasticity of the matrix, dissimilarity of the platelets and non-uniform shear distributions in the overlap region ( Supplementary Fig. 5 ). As shown in Fig. 5 , stiffness changes minimally with varying ξ and is not a function of C . Strength gets larger as the degree of plasticity increases and saturates slower as ξ decreases. Figure 5e,f shows that toughness is maximized for composites with uniformly staggered platelets ( ξ =0.5). However, as λL →∞, stiffness, strength and toughness of composites with varying ξ approach those of ξ =0.5, in line with common intuition that both ξ λ L and (1– ξ ) λL become infinite as λL →∞. Universal composition–structure–property maps Having fully characterized the elastic and elastic-perfectly plastic responses of the composite within a non-uniform staggering distribution of platelets, here we aim at developing a unified map decoding the non-intuitive synergies between structures and materials that confer mutually inclusive or exclusive mechanical properties in the generalized platelet–matrix composite. In view of Fig. 1e ( C =0 and ξ =0.5), to effectively obtain the maximum strength capacity of the unit cell for each specific k , we define the composite ‘strong’ if its characteristic overlap length, λL , is equal or larger than a critical value, λL cr , at which the normalized strength has reached at least 90% of its saturation value (black dots in Fig. 1e ). This definition does not imply that composites with λL < λL cr are not strong; instead, it means that they have not yet utilized their maximum theoretical capacities. The blue inset in Fig. 1e clearly illustrates this definition in a 2D diagram for all values of k and relevant λL cr . As k increases, the normalized strength requires a larger λL cr to reach its respective 90% of the upper limit. Hence, given the platelet elastic moduli, width ratios ( k ) and interface properties ( λ ), this diagram identifies the minimum required platelet length to make a strong composite that can exhibit at least 90% of its maximum theoretical strength capacity, . Similarly, we consider the unit cell ‘tough’ for any given k if its λL in Fig. 1f is within a critical range for which the normalized toughness is at least 90% of its maximum theoretical capacity, . In Fig. 1f , the parameters and 90% are represented by dashed and solid lines, respectively, and the yellow diagram in the inset demonstrates the ‘tough’ region for all values of k . Analogous to the definition of ‘strong’, we consider the unit cell ‘stiff’ for any given k if its λL in Fig. 1g is equal or larger than a critical value, λL cr , for which the normalized stiffness is at least 90% of its maximum theoretical capacity, . Finally, by overlapping insets of Fig. 1e–g , and extending the above analysis to various degrees of matrix plasticity ( C ≠0) and various platelet offset ratios ( ξ ≠0.5), we construct a set of universal diagrams representing normalized strength, toughness and stiffness in the space of ( λL , k ) applicable to all natural and biomimetic platelet–matrix composites and stacked heterostructures ( Fig. 6 ). 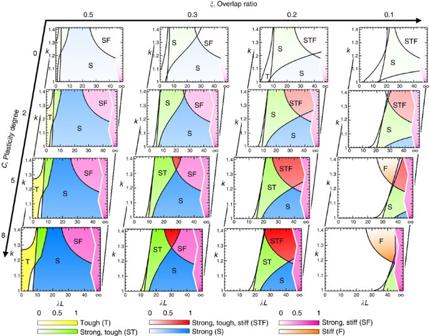Figure 6: Universal composition–structure–property maps. The coloured regions correspond to optimum mechanical properties, which are inclusively/exclusively strong (S), tough (T) and/or stiff (F) depending on the value of characteristic length (λL), platelet dissimilarity (k), matrix plasticity (C) and platelet overlap offset ratio (ξ). For a given (k,C,ξ), the borderlines correspond to a criticalλL, for which a property (for example, T) or a set of properties (e.g., ST) is 90% of its maximum theoretical capacity. Given the values of the universal dimensionless quadruple (λL,k,C,ξ), one can readily determine to what extent the material has attained or sanctified its mutually exclusive (inclusive) mechanical properties. The intensity of the colours represents the relative value of the properties. To predict the absolute values of the properties, see text. Compared withξ, the increase inCmainly accounts for increased absolute values of the properties with relatively small changes in the boundaries. On the other hand, the increase in offset ratio (ξ→0) results in small alterations in absolutes values (compared with the effect ofC) but significant changes in the boundaries of overlapping regions, particularly enabling overlapping optimum properties for composites with dissimilar platelets. The advantage of such diagrams is that one can map all the important structural, material and mechanical information (both in terms of overlapping optimum properties and their relative values) in simple 2D plots and infer the following: Figure 6: Universal composition–structure–property maps. The coloured regions correspond to optimum mechanical properties, which are inclusively/exclusively strong (S), tough (T) and/or stiff (F) depending on the value of characteristic length ( λL ), platelet dissimilarity ( k ), matrix plasticity ( C ) and platelet overlap offset ratio ( ξ ). For a given ( k , C , ξ ), the borderlines correspond to a critical λL , for which a property (for example, T) or a set of properties (e.g., ST) is 90% of its maximum theoretical capacity. Given the values of the universal dimensionless quadruple ( λL , k , C , ξ ), one can readily determine to what extent the material has attained or sanctified its mutually exclusive (inclusive) mechanical properties. The intensity of the colours represents the relative value of the properties. To predict the absolute values of the properties, see text. Compared with ξ , the increase in C mainly accounts for increased absolute values of the properties with relatively small changes in the boundaries. On the other hand, the increase in offset ratio ( ξ →0) results in small alterations in absolutes values (compared with the effect of C ) but significant changes in the boundaries of overlapping regions, particularly enabling overlapping optimum properties for composites with dissimilar platelets . Full size image Given a ( λL , k ) pair, a platelet–matrix composite may be inclusively/exclusively strong, tough (in the context of intrinsic toughening mechanisms) and/or stiff depending on the degree of matrix plasticity ( C ) and overlap offset ratio ( ξ ). Generally speaking, compared with the effect of offset ratio ( ξ ), the increase in matrix plasticity ( C ) mainly accounts for increased absolute values of the strength and toughness with relatively small changes in the boundaries of overlapping region. On the other hand, the increase in offset ratio ( ξ →0)—for a constant matrix plasticity ( C )—results in small alterations in absolutes values (compared with the effect of plasticity) but significant changes in the boundaries of overlapping regions, particularly enabling overlapping optimum properties for composites with dissimilar platelets . While strength and stiffness exhibit similar trend versus λL (both saturate with λL ), stiffness saturation happens at a much slower pace than strength, especially for platelets with large stiffness and/or thickness contrasts ( k →1). However, as ξ →0 and/or C increases, the critical characteristic length ( λL cr ) of strength moves to the right, thus increasing the chance of overlap between the optimally strong and stiff regions, or even strong, tough and stiff regions. Contrary to stiffness and strength, toughness maximizes at a finite λL. Increasing matrix plasticity and/or offset ratio increases the characteristic length ( λL cr ) of toughness and also widens the range of this λL cr , thereby increasing the chance of finding an overlapping region where strength, toughness and stiffness are balanced. The white areas in Fig. 6 are physically admissible but indicate that the composite has not yet exhibited its optimum toughness and/or strength capacities. The quadruple λL , k , C and ξ are dimensionless universal characteristic parameters, making their absolute values and their interplays (borderlines) in Fig. 6 applicable to all generalized platelet–matrix composites made of similar and/or dissimilar platelets. This is a critical advantage of these diagrams and the significant result of this paper, which can be used as a guiding toolbox for knowledge-based synthesis of numerous biomimetic composites and stacked heterostructures. The intensity of the colours in Fig. 6 represents the relative values of the properties. For overlapping regions (for example, tough and strong), the colour intensity is the arithmetic average of the relative overlapping properties. Although approximated (that is, distinct mechanical properties cannot be added together), Fig. 6 qualitatively predicts the relative values of the optimum mechanical properties in the space of ( λL , k , C , ξ ). To predict the absolute value of the properties, one can take the optimum ( λL , k ) in Fig. 6 and plug them into Fig. 5 to read (interpolate) the normalized values of the properties for a given ( C , ξ ) and then simply obtain the absolute values by multiplying them to the normalization factors. Alternatively, one can directly plug the optimum ( λL , k ) into Supplementary equations (73), (75) and (77) to obtain the exact absolute values of stiffness, strength and toughness, respectively. In essence, the borderlines in diagrams of Fig. 6 represent whether the generalized platelet–matrix composite is able to achieve the maximum capacity for a certain property (or a set of properties) given the space of ( λL , k , C , ξ), and the intensity of the colours represents the relative normalized values of the mechanical properties. To better understand these features and test our results, Fig. 7 shows the diagram with C =0 and ξ =0.5 that is superimposed with the 12 ( λL , k ) pairs of our 3D-printed specimens, validating our predicted theoretical capacities vis-à-vis experiments ( Supplementary Table 2 ). For instance, specimen c lies in the green region of Fig. 7 indicating optimum strength and toughness; in accord with the highest measured and . 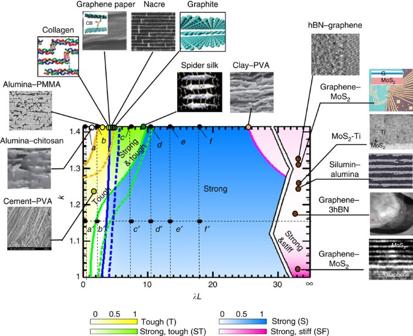Figure 7: Overlay of composition–structure–property diagram with natural and biomimetic composites. The lines (for elastic composites withC=0) and dash lines (for plastic composites withC=2) correspond to the criticalλL, defining the boundaries of achieving 90% of strength (blue line), toughness (orange and green lines) and stiffness (magenta line). These lines move to the right as plasticity increases. Intensity of the colours shows the relative values of the properties forC=0. To predict the absolute values of the properties, see text. The (k,λL) parameters are universal dimensionless parameters, thus their absolute values are applicable to many real platelet–matrix composites and stacked heterostructures. This important feature is evident from overlaying several natural and biomimetic platelet–matrix composites as well as stacked heterostructures onto the above diagram. This is a significant result of this paper and can be used as a guiding toolbox for knowledge-based synthesis of numerous biomimetic composites as well as emerging heterostructures. The letters corresponds to the 3D-printed specimens. The predicted locations of these specimens match with their experimentally measured properties. The (λL,k) data of natural and synthetic platelet–matrix composites and stacked heterostructures are calculated from the literature7,9,10,21,22,23,25,27,28,33,43,44,45,46,47,48,49,50,51,52,53,54,55,56. Snapshots of the natural and biomimetic composites are adapted with permission from ref.20Copyright 2012 American Chemical Society, adapted with permission from ref.23Copyright 2012 American Chemical Society and adapted with permission from refs9,10,21,22,25,33,57,58. PMMA, poly(methyl methacrylate). Figure 7: Overlay of composition–structure–property diagram with natural and biomimetic composites. The lines (for elastic composites with C =0) and dash lines (for plastic composites with C =2) correspond to the critical λL , defining the boundaries of achieving 90% of strength (blue line), toughness (orange and green lines) and stiffness (magenta line). These lines move to the right as plasticity increases. Intensity of the colours shows the relative values of the properties for C =0. To predict the absolute values of the properties, see text. The ( k , λL ) parameters are universal dimensionless parameters, thus their absolute values are applicable to many real platelet–matrix composites and stacked heterostructures. This important feature is evident from overlaying several natural and biomimetic platelet–matrix composites as well as stacked heterostructures onto the above diagram. This is a significant result of this paper and can be used as a guiding toolbox for knowledge-based synthesis of numerous biomimetic composites as well as emerging heterostructures. The letters corresponds to the 3D-printed specimens. The predicted locations of these specimens match with their experimentally measured properties. The ( λL , k ) data of natural and synthetic platelet–matrix composites and stacked heterostructures are calculated from the literature [7] , [9] , [10] , [21] , [22] , [23] , [25] , [27] , [28] , [33] , [43] , [44] , [45] , [46] , [47] , [48] , [49] , [50] , [51] , [52] , [53] , [54] , [55] , [56] . Snapshots of the natural and biomimetic composites are adapted with permission from ref. 20 Copyright 2012 American Chemical Society, adapted with permission from ref. 23 Copyright 2012 American Chemical Society and adapted with permission from refs 9 , 10 , 21 , 22 , 25 , 33 , 57 , 58 . PMMA, poly(methyl methacrylate). Full size image To demonstrate the universality of the composition–structure–property maps in Fig. 6 , we overlaid the diagram with ξ =0.5 with several existing natural and biomimetic platelet–matrix composites as well as stacked heterostructures and let C go from 0 to 2, representing fully elastic and 200% plastic matrix ( Fig. 7 ). We used the uniform ( ξ =0.5), versus non-uniform, staggering since ξ ≠0.5 leads to lower mechanical properties (see Fig. 5 ), thus likely less common staggering pattern for a general description of natural and biomimetic composites and stacked heterostructures. Then, by calculating the ( λL , k ) pairs for a wide range of materials with geometrical and material characteristics from atomic scale to microscale ( Supplementary Table 1 ), we identified their precise locations in Fig. 7 . For example, nacre, consisting of platelets of a few hundred nanometres to micrometre dimensions , and silk, consisting of platelets of nanometre range , lie in the ‘strong, tough’ regions, consistent with the previous studies [32] , [33] . By mimicking nacre, nanoscale clay–PVA (polyvinyl alcohol) composites are reported to be ultrastrong and stiff [9] , consistent with the ‘stiff and strong’ region of the diagram of Fig. 7 . The universality of the map of Fig. 7 can be also verified with composites made of dissimilar platelets. For instance, a bilayer cement-PVA nanocomposite connected by a network of hydrogen bonds has been shown to exhibit high toughness but at the expense of lower strength than the maximum capacity [28] , consistent with the prediction of Fig. 7 ( λL =1.7, k =1.251). Stacked heterostructures such as h-BN-graphene or graphene-MoS 2 are another important class of composites, which are composed of dissimilar platelets with strong in-plane bonding networks but weak interplanar van der Waals bonding matrices. Although there are no experimentally measured values (to our knowledge) on the composite strength, stiffness and toughness values of such heterostructures, Fig. 7 predicts these composite structures to be on the right extreme, that is, ‘stiff and strong’, owing mainly to the high stiffness of the platelets and large overlap domain ( λL ≥26). However, by reducing λL , for example, via lowering the overlap length, these multifunctional stacked heterostructures can even exhibit toughness, thereby preventing or hampering their typical brittle fracture. Note that the solid borderlines of various optimum properties in Fig. 7 corresponds to elastic response ( C =0). By considering the plasticity of the matrix, these borderlines typically move to the right of the diagram. As an example, the dashed lines in Fig. 7 corresponds to C =2 (200% ratio of the plastic to elastic strain), which are easily distinguishable compared with C =0. One can also use this strategy to further include extrinsic and hierarchical toughening mechanisms, and interlocking phenomena in Fig. 7 and quantify the relative values and locate the positions of the modified borderlines with respect to the intrinsic toughening mechanisms. Platelet and/or matrix failure So far our analyses were based on matrix failure. If the platelets are not strong enough, the composite might fail from the platelets before the matrix reaches the maximum shear stress. Let represent the ratio of the strength of the top and bottom platelets, respectively, to the yielding strength of the matrix, τ f , that is, . Then, under platelets and/or matrix failures, the effective strength and toughness of the generalized platelet–matrix composite with an elastic-perfectly plastic matrix and offset overlap ratio can be written as In equation (8), ϕ =min{ ϕ 1 , ϕ 2 } and is the normalized composite strength under matrix failure including the effect of matrix plasticity. 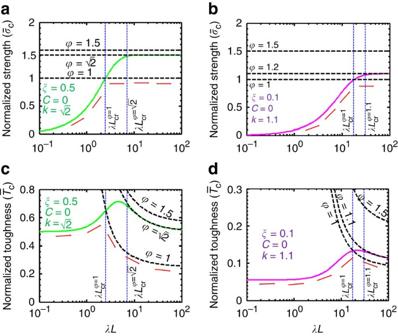Figure 8: Mechanical properties considering both matrix and platelet failures. (a,b) Normalized strength,, (c,d) Normalized toughness,for an elastic platelet–matrix composite. (a,c) correspond to composites with identical platelets and no overlap offset. (b,d) represent an example of a composite with dissimilar platelets and overlap offset ratio. Toughness under platelet failure varies withλL,k,Candξ. The coloured solid lines (green forξ=0.5 and magenta forξ=0.1) show toughness and strength based on matrix failure. The black dashed lines denote toughness and strength under platelet failure scenarios for different ratios of platelet to matrix strengths, represented byϕ. The blue dashed lines showλLat which the platelet and the matrix fail simultaneously. The red arrows show an example (forϕ=1) path of ultimate toughness and strength versusλL, which is equal to the minimum of toughness and strength values based on both the matrix and platelet failures. Figure 8 illustrates the behaviour of equation (8) versus λL for various values of ϕ , and also the conditions at which the platelet and the matrix fail simultaneously. For example, considering strength, the following criteria clearly describes the matrix and/or platelets failure mechanisms (see also Fig. 5c,d ) Figure 8: Mechanical properties considering both matrix and platelet failures. ( a , b ) Normalized strength, , ( c , d ) Normalized toughness, for an elastic platelet–matrix composite. ( a , c ) correspond to composites with identical platelets and no overlap offset. ( b , d ) represent an example of a composite with dissimilar platelets and overlap offset ratio. Toughness under platelet failure varies with λL , k , C and ξ . The coloured solid lines (green for ξ =0.5 and magenta for ξ =0.1) show toughness and strength based on matrix failure. The black dashed lines denote toughness and strength under platelet failure scenarios for different ratios of platelet to matrix strengths, represented by ϕ . The blue dashed lines show λL at which the platelet and the matrix fail simultaneously. The red arrows show an example (for ϕ =1) path of ultimate toughness and strength versus λL , which is equal to the minimum of toughness and strength values based on both the matrix and platelet failures. Full size image For toughness, the situation is more complex depending on ( λL , k , C , ξ ). In essence, the ultimate value of strength (toughness) for varying λL is the minimum of strength (toughness) under the matrix and/or platelet failures. This is represented by red arrows (for the example of ϕ =1) in Fig. 8 , which show the path of toughness and strength versus λL considering platelet and/or matrix failures. These analyses are further extended to include platelet failures when considering stairwise and random staggering distribution of the platelets and our results indicate that while the former may improve the composite properties, the latter typically lead to lower mechanical properties ( Supplementary Figs 6–9 ). Nevertheless, a rough estimation based on σ f =0.1 E and τ f =0.1 G and assuming a large plasticity of the matrix (that is, C =8) shows that in majority of the natural and synthetic platelet–matrix composites and stacked heterostructures , indicating that the matrix failure is dominant ( Supplementary Table 4 ). We also obtained the detailed stress–strain trajectories, demonstrating more insights into the transitions from linear elasticity to one- and/or two-sided plasticity, to full plasticity and eventually rupture ( Fig. 9 , Supplementary Figs 10 and 11 ). 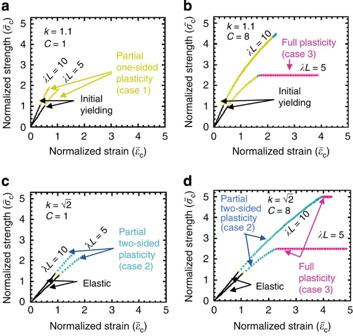Figure 9: Trajectories of stress–strains. (a–d) Stress–strainplots of composites for differentk,CandλL(in all cases,ξ=0.5). Each figure includes two plots forλL=10 (top) andλL=5 (bottom). Different colours show different stages of matrix deformation in the composite: black (elastic), gold (partial one-sided plasticity, case 1), blue (partial two-sided plasticity, case 2) and magenta (full plasticity, case 3). Figure 9: Trajectories of stress–strains. ( a – d ) Stress –strain plots of composites for different k , C and λL (in all cases, ξ =0.5). Each figure includes two plots for λL =10 (top) and λL =5 (bottom). Different colours show different stages of matrix deformation in the composite: black (elastic), gold (partial one-sided plasticity, case 1), blue (partial two-sided plasticity, case 2) and magenta (full plasticity, case 3). Full size image The key novelty of this work lies in reducing the complexity and non-intuitive synergies of the platelet–matrix systems to a few (four) universal dimensionless parameters and in providing guidelines as to how these universal characteristic parameters can be modulated to optimize conflicting mechanical properties of such composites. From this perspective, the condensation of our results in the form of ‘Universal Composition–Structure–Property Design maps’, containing only four characteristic parameters, is a significant first step in the field, which places the platelet–matrix composites in equal footing with nanocrystalline metallic systems and alloys in the current applications of structure–property relationships to significantly alter the material design landscape. Broadly, the innovative concepts, strategies and techniques of this work (specially the notion of universal maps), although casted in the context of platelet–matrix architectures, have important implications for understanding and mimicking several other fascinating damage-tolerant natural composites, which are similarly made of hard and soft building blocks but arranged in different architectures (for example, criss-cross decussation in tooth enamel [34] , Bouligand arrangement in exoskeleton of anthropod [2] , helicoidal matrix of hammer-like dactyl clubs of the stomatopods [35] and so on). Furthermore, one can employ the novel concept and strategies of this work to create universal design maps for other synthetic material classes such as cermets, metallic glasses, combinatorial and particulate oxides, boron nitride layered composites and emerging high entropy alloys [36] , [37] , [38] , [39] , [40] , [41] , [42] . This work proposes a new dimensionless characteristic quadruple, ( λL , k , C , ξ ), to quantify the stiffness, strength and toughness of platelets-matrix composites and stacked heterostructures with an elastic and elastic-perfectly plastic matrices as well as platelets with non-uniform staggering distributions. Given the value of ( λL , k , C , ξ), one can readily determine to what extent the composite has attained or sacrificed its mutually exclusive (inclusive) mechanical properties and also readily predict the absolute values of the mechanical properties. By mapping an extensive range of λL , k , C , ξ values into a set of 2D diagrams, we constructed a universal framework that offers a simple, yet powerful tool to decode the non-intuitive synergies between structures, materials and properties of generalized platelet–matrix composites. Validated by several 3D-printed specimens, and a wide spectrum of existing natural and biomimetic composites as well as stacked heterostructures across different scales and material classes, the proposed diagrams provide a deep understanding on how to intelligently utilize the maximum theoretical capacities for simultaneously improving strength, toughness and/or stiffness, and to design new heterostructures and platelet–matrix composites with contrasting platelet characteristics. This work opens up several new opportunities to further extend the proposed diagrams to include and quantify the effect of locking mechanisms [43] , stacked multi-heterostructures [22] , extrinsic and hierarchical toughening processes [31] and so on and identify new boundaries and overlaps in multi-phase multi-functional materials. Synthesis All specimens used in the study were printed at Stratasys, in Minnesota, USA using an Objet Connex500 multi-material 3D printer. In a single print, we fabricated composites made of two base materials with strongly contrasting material properties ( Fig. 3a ). All platelets were made of VeroWhitePlus, while the matrices were made of either TangoBlackPlus 27ShoreA (for specimens a,a′,b,b′ ) or TangoBlack 95ShoreA (for the rest). These materials are all proprietary acrylic-based photopolymer, and we will henceforth refer to them as Material A, Material B and Material C, respectively. In all specimens, the lighter phase represents the stiffer constituent and was printed with Material A, and the darker phase, representing the compliant constituent, was printed with Material B or C. Figure 3a indicates the relative planar dimensions of the test specimens and Supplementary Table 1 shows all the detailed structural dimensions. To print the composites, we used a dual material jetting technology allowing two distinct materials to be printed simultaneously. Each material resides in cartridges and is funneled through a liquid system that is connected to the printing block consisting of eight printing heads. Two printing heads, each containing 96 nozzles with 50 μm diameters, are used for printing each of the two base materials, while the remaining printing heads are reserved for printing a support material. An ultraviolet light follows the printing heads to immediately cure the printed materials, thus letting new layers to be printed instantaneously. We printed 12 specimens covering a wide range of overlap lengths and width ratios as detailed in Supplementary Table 1 . Owing to an in situ curing of the printed materials, the Materials A and B (and A and C) adhere to each other perfectly, that is, no interfacial debonding or sliding on loading, consistent with our theory and confirmed by the experiments ( Supplementary Movie 1 ). To avoid undesirable bending, and ensure pure shear deformations in the matrix and axial deformations in the platelets, we printed symmetric specimens by mirroring the unit cells as shown in Supplementary Fig. 3 . In view of the definition of , the platelet contrast can be introduced via m or n or both. Owing to the current limitation of the dual material jetting technology, which can print only two materials at a time, we introduced platelet contrast via varying the width ratios of the platelets ( m ) while using identical material (Material A) for all platelets, that is, constant n ( Supplementary Table 1 ). Tensile experiments For optimal griping of the specimens in the tensile testing apparatus, we attached (printed) two small uniform strips, made of Material A, to the two ends of the specimens ( Supplementary Fig. 3 ). We tested the 3D-printed specimens in an Instron 4500 Universal Testing Machine with a 100-kN static load cell and applied displacement boundary conditions until failure. The load capacity of the grips is 100 kN and the spring stiffness of the entire testing device far exceeds the stiffness of our specimens. We attached our specimens firmly in the grips and centre the middle platelet of the geometries with the force applied through the vice action grips to ensure pure shear in the matrix and axial deformations in the platelets. We did this to emulate the boundary conditions applied in our theoretical derivations. In the tensile test, we employed a displacement rate of 2.5 mm min −1 . Base materials Selections of various Objet printable materials with different bulk mechanical properties are already available. The referenced data of Stratasys indicates that of the materials available for printing, the three employed in this study represent a strong contrasting mechanical behaviour: Materials A being the hardest, Material B being the softest and Material C being slightly stiffer that Material B. However, there is no previous data on the shear modulus, G , of these materials or the interfacial shear strength, τ f , between them. To obtain G and τ f for the platelet–matrix system of A–B, we fabricated three identical test specimens similar to the specimen ‘ a ’ but with a short overlap length (3 cm) to have (almost) uniform shear along the overlap length ( Fig. 2 ). Next via straining the specimens with the same procedure as detailed above, we obtained the force–displacement ( F − δ ) plots. Then, the shear modulus of Material B and interfacial shear strength of the A–B interface were approximated by and , respectively. Using a similar procedure, we found G =6.73±0.28 MPa and τ f =6.93±0.3 MPa for the Material C and the A–C interface, respectively. The Young modulus of Material A ( E 1 ) is reported to be 2.50±0.5 GPa from the manufacturer and was used in this study. The modulus of the most compliant material, B, is three orders of magnitude lower than the stiffer material, A, by a factor of ≈ 1900. In view of this large factor, we only considered the uncertainty in the E 1 as the source of error bars. See Supplementary Note 1 for analysis of elastic deformations, Supplementary Note 2 for details on composite stiffness, Supplementary Table 1 , Supplementary Note 3 and Supplementary Figs 1–3 for experimental details, Supplementary Note 4 for analysis of plastic deformations, Supplementary Note 5 and 6 for studying the effects of overlap offset, Supplementary Note 7 for studying platelet versus matrix failures, Supplementary Note 8 and 9 for analysis of stairwise and random staggering, Supplementary Note 10 for derivation of stress–strain plots, Supplementary Note 11 and Supplementary Fig. 12 for analysis of volume fraction. How to cite this article: Sakhavand, N. and Shahsavari, R. Universal composition–structure–property maps for natural and biomimetic platelet–matrix composites and stacked heterostructures. Nat. Commun. 6:6523 doi: 10.1038/ncomms7523 (2015).